ABA signalling is fine-tuned by antagonistic HAB1 variants Group A protein type 2C phosphatases (PP2Cs) are negative regulators of abscisic acid (ABA) signalling and plant adaptation to stress. However, our knowledge of the regulation of PP2C activity is limited. Here we report that the PP2C HAB1 undergoes alternative splicing to produce two splice variants, which encode HAB1.1 and HAB1.2, that play opposing roles in ABA-mediated seed germination and ABA-mediated post-germination developmental arrest. HAB1.2 is predominately formed in the presence of ABA and prevents seed germination and post-germinative growth. HAB1.2 interacts with OST1, but cannot inhibit OST1 kinase activity; thus, it functions as a positive regulator of ABA signalling. We also identified an RNA-recognition motif-containing protein, RBM25, as a potential regulator of HAB1 alternative splicing and molecular diversity. Our results reveal a mechanism for turning ABA signalling on and off and for plant adaptation to abiotic stress. Abscisic acid (ABA) is essential for plant adaptation to abiotic stresses, such as drought [1] , [2] , [3] , [4] . The identification of the PYR/PYLs/RCAR protein family (hereafter referred to as PYLs) as ABA receptors has led to a breakthrough in ABA signalling. In the absence of ABA, group A protein type 2C phosphatases (PP2Cs) interact with subclass III SNF1-related protein kinases (SnRK2.2, 2.3 and 2.6) to dephosphorylate and inhibit their kinase activity and turn off ABA signalling. ABA binds to PYLs, promoting their interaction with PP2Cs and inhibiting their phosphatase activity [5] , [6] , [7] . Thus, SnRK2s are released from PP2C–SnRK2 complexes to phosphorylate downstream effectors and activate ABA signalling [3] , [5] , [6] , [8] , [9] , [10] . Over the past several years, the structures and molecular functions of ABA receptors have received significant attention [9] , [10] , [11] . PP2Cs are central components of the core PYL–PP2C–SnRK2 regulatory module [1] . However, our knowledge of the activity of PP2Cs is poor, limiting our understanding of ABA signalling and plant adaptation to stress. In Arabidopsis , nine group A PP2Cs interact with PYLs in the presence of ABA [5] , [11] , [12] , [13] , [14] . HAB1 is among the best-characterized PP2Cs in ABA signalling [15] . HAB1 is broadly expressed in various tissues and organs and is induced by ABA treatment [16] . HAB1 binds to and dephosphorylates SnRK2s, especially SnRK2.6 (OST1), and negatively regulates ABA signalling [17] , [18] . Genetic analyses have suggested that HAB1 is functionally redundant with ABI1 and ABI2 in the regulation of post-germination development and stomatal movement under drought conditions [19] , [20] . It is apparent that HAB1 is essential in ABA signalling. Therefore, accurate regulation of HAB1 expression and phosphatase activity is required for the fine-tuning of ABA signalling and plant adaptation to stress. The removal of introns from intron-containing genes through the splicing of pre-mRNAs is emerging as a key step in gene expression [21] , [22] . Alternative splicing (AS) regulates not only transcript levels but also transcript isoforms, giving rise to proteins that differ in subcellular localization, stability and function [23] , [24] , [25] . More than 61% of intron-containing Arabidopsis genes undergo AS under normal conditions [26] . The percentage of genes showing AS will dramatically increase when plants are subjected to abiotic stresses. Thus, AS plays a fundamental role in plant development and stress adaptation [27] , [28] . We are beginning to understand the potential control of AS over hormone signalling [23] , [25] . However, the role of AS in regulating ABA signalling and plant stress adaptations remains elusive. A bioinformatic analysis predicted that all nine group A PP2C transcripts contain introns, and among them HAB1 and ABI2 may be subject to AS. Do PP2C transcripts undergo AS? If so, what is the functional consequence in terms of the regulation of ABA signalling? Further, how is the selection of alternatively spliced isoforms regulated? To address these important questions, we analysed the transcripts of nine PP2Cs . Of these nine we only detect two splice variants from HAB1 , HAB1.1 and HAB1.2. We also provide evidence showing that HAB1.2 and HAB1.1 have opposing functions in ABA signalling. Moreover, the HAB1.2/HAB1.1 ratio is an important on–off switch in ABA signalling and plant responses to ABA. We also demonstrate that an RNA-binding motif (RBM)-containing protein RBM 25, a homologue of HsRBM25, is a potential key regulator of HAB1 AS in Arabidopsis . Our results provide important and novel insight into the regulation of HAB1 expression and activity and into the complex regulation of ABA signalling. HAB1 undergoes ABA-controlled AS during early development To analyse whether group A PP2C transcripts are subjected to AS in response to ABA, we first performed RT–PCR using three primer pairs per gene with 7-day-old wild-type seedlings treated with or without ABA. Our results indicate that HAB1 has two transcripts regardless of ABA treatment in the young seedlings ( Supplementary Fig. 1 ). Our results also indicate the production of two splice variants of HAB1 during seed germination and post-germination development under normal conditions ( Fig. 1a ). Because the HAB1 locus consists of four exons and three introns ( Fig. 1b ), the above result led us to speculate that HAB1 is subjected to AS. Sequencing confirmed that the lower band was full-length HAB1 ( HAB1.1 ) encoding a HAB1 protein (HAB1.1) with 511 amino acids, whereas the upper band was an alternatively spliced variant of HAB1 , HAB1.2 , containing the third intron, a cryptic exon of 123 nucleotides ( Fig. 1b ). However, HAB1.2 encodes a smaller (416 amino acid) protein, HAB1.2, lacking the C-terminal 105 amino acids because of a premature stop codon ( Fig. 1b and Supplementary Fig. 2a ). Bioinformatic predictions from TAIR support the existence of HAB1 splice variants ( Supplementary Fig. 2b ). 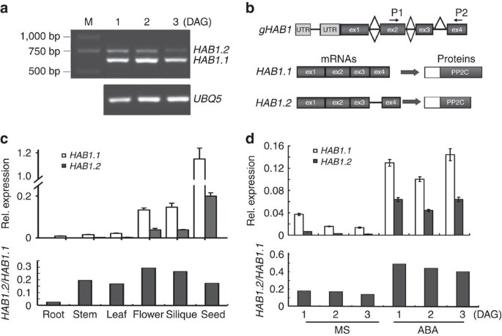Figure 1: Alternative splicing ofHAB1. (a) RT–PCR analysis of theHAB1transcript levels at 1, 2 and 3 days after germination. ‘M’ indicates DNA molecular weight ladder. (b) Schematic diagram outlining the organization of theHAB1.1andHAB1.2variants. The primers used in theaare indicated as P1 and P2. (c) qRT–PCR analysis of theHAB1variants in different tissues. (d) qRT–PCR analysis of theHAB1variants at 1, 2 and 3 days after germination with or without 100 μM ABA treatment for 3 h in wild type.GAPDHwas used as an internal control. The values were normalized to that ofGAPDH. The s.d. of three technical replicates is shown using error bars. Three biological replicates were performed and each gave the similar result. Figure 1: Alternative splicing of HAB1 . ( a ) RT–PCR analysis of the HAB1 transcript levels at 1, 2 and 3 days after germination. ‘M’ indicates DNA molecular weight ladder. ( b ) Schematic diagram outlining the organization of the HAB1.1 and HAB1.2 variants. The primers used in the a are indicated as P1 and P2. ( c ) qRT–PCR analysis of the HAB1 variants in different tissues. ( d ) qRT–PCR analysis of the HAB1 variants at 1, 2 and 3 days after germination with or without 100 μM ABA treatment for 3 h in wild type. GAPDH was used as an internal control. The values were normalized to that of GAPDH . The s.d. of three technical replicates is shown using error bars. Three biological replicates were performed and each gave the similar result. Full size image Next, we investigated whether HAB1 AS occurs during other developmental stages using primers surrounding the region of each HAB1 variant for quantitative quantitative reverse transcriptase–PCR (qRT–PCR). As shown in Fig. 1c , very low levels of HAB1.1 and HAB1.2 transcripts were detected in the roots of young seedlings. The expression of HAB1.1 and HAB1.2 was markedly increased in flowers and siliques, and reached its highest level in seeds. However, HAB1.1 and HAB1.2 were detected at a similar ratio in all tested tissues, except roots ( Fig. 1c ). It has been shown that HAB1 plays a key role in the post-germination developmental arrest induced by ABA [16] . To understand the role of HAB1 AS in early plant development, we examined the expression of the two variants and the effects of ABA on HAB1 AS. In the absence of ABA, both HAB1.1 and HAB1.2 were detected in germinating seeds, but the HAB1.2 transcript level was much lower than the HAB1.1 transcript level ( Fig. 1d ). The transcript levels of HAB1.1 and HAB1.2 were decreased within 3 days of germination after stratification with a relatively low ratio (0.17) of HAB1.2 to HAB1.1 ( Fig. 1d ). Intriguingly, in the presence of ABA, the HAB1.1 and HAB1.2 transcripts were substantially upregulated and maintained at high levels throughout germination and cotyledon greening ( Fig. 1d ). Notably, HAB1.2 showed a greater increase than HAB1.1 , resulting in an increased HAB1.2 / HAB1.1 ratio. These results suggest a role of HAB1.2 in ABA-triggered delayed seed germination and the post-germination developmental arrest. HAB1 variants have opposite functions in ABA sensitivity Because HAB1.1 is a negative regulator of ABA signalling, and given that a loss of function or overexpression of HAB1.1 results in ABA-hypersensitive or -insensitive phenotypes during germination and post germination, respectively [16] , we investigated the function of HAB1.2 in the ABA response during early development. We generated transgenic plants overexpressing c-Myc-tagged recombinant HAB1.2 protein in a HAB1 loss-of-function mutant, hab1-1 . To achieve HAB1.2 overexpression, we created two point mutations at the 5′ splice site (from Gg to At) in the third intron to produce HAB1.2pm , which allowed retention of the third intron in the transcript ( Fig. 2a ). We then performed RT–PCR and western blot analysis and found that HAB1.2 was successfully expressed and translated into protein ( Fig. 2b,c ). 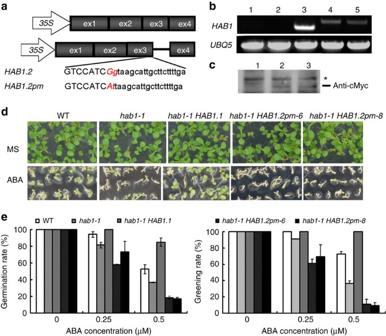Figure 2: TheHAB1variants have opposing functions in the plant ABA response. (a) Schematic diagram showing the constructs used to overexpressHAB1.1andHAB1.2. The mutated nucleotides are marked in red. (b) RT–PCR analysis to detect the overexpression ofHAB1.1orHAB1.2in the transgenic lines. RNA was isolated from 7-day-old seedlings. Lane 1: wild type; lane 2:hab1-1; lane 3:hab1-1HAB1.1; lane 4:hab1-1HAB1.2-6; lane 5:hab1-1HAB1.2-8.(c) Western blot analysis of HAB1.2 expression in the transgenic linehab1-1HAB1.2. Total protein was extracted from 7-day-old seedlings, and HAB1.2 was detected using anti-myc antibodies; the star indicates unspecific binding. Lane 1: wild type; lane 2:hab1-1HAB1.2-6; lane 3:hab1-1HAB1.2-8.(d) Seed germination and the development of wild-type,hab1-1,hab1-1HAB1.1,hab1-1HAB1.2-6andhab1-1HAB1.2-8plants on MS medium with or without 0.5 μM ABA. The pictures were taken 8 days after germination. (e) Comparison of the germination rates for 5-day-old seedlings (left) and the greening rates for 8-day-old seedlings (right) treated with or without ABA. The s.d. of three experiments is shown using error bars. Figure 2: The HAB1 variants have opposing functions in the plant ABA response. ( a ) Schematic diagram showing the constructs used to overexpress HAB1.1 and HAB1.2 . The mutated nucleotides are marked in red. ( b ) RT–PCR analysis to detect the overexpression of HAB1.1 or HAB1.2 in the transgenic lines. RNA was isolated from 7-day-old seedlings. Lane 1: wild type; lane 2: hab1-1 ; lane 3: hab1-1HAB1.1 ; lane 4: hab1-1HAB1.2-6 ; lane 5: hab1-1HAB1.2-8. ( c ) Western blot analysis of HAB1.2 expression in the transgenic line hab1-1HAB1.2 . Total protein was extracted from 7-day-old seedlings, and HAB1.2 was detected using anti-myc antibodies; the star indicates unspecific binding. Lane 1: wild type; lane 2: hab1-1HAB1.2-6 ; lane 3: hab1-1HAB1.2-8. ( d ) Seed germination and the development of wild-type, hab1-1 , hab1-1HAB1.1 , hab1-1HAB1.2-6 and hab1-1HAB1.2-8 plants on MS medium with or without 0.5 μM ABA. The pictures were taken 8 days after germination. ( e ) Comparison of the germination rates for 5-day-old seedlings (left) and the greening rates for 8-day-old seedlings (right) treated with or without ABA. The s.d. of three experiments is shown using error bars. Full size image Next, we characterized the ABA response of hab1-1HAB1.2pm homozygous plants using wild type, hab1-1 - and hab1-1 -overexpressing HAB1.1 as controls ( Fig. 2d,e ). In the absence of ABA, seed germination and cotyledon greening in the hab1-1HAB1.2pm transgenic plants were comparable to that in wild type, hab1-1 and hab1-1HAB1.1 ( Fig. 2d,e ). When germinated on a medium containing various concentrations of ABA, hab1-1 and hab1-1HAB1.1 plants were more sensitive or more tolerant to ABA than wild type during both the germination and greening stages, respectively ( Fig. 2d,e ), in accordance with previous findings [16] . In sharp contrast, the hab1-1HAB1.2pm plants exhibited greater ABA sensitivity than hab1-1 ( Fig. 2d,e ). For example, in the presence of 0.5 μM ABA, the germination rate of hab1-1HAB1.2pm was reduced by ∼ 50% compared with the hab1-1 mutant, while the percentage of hab1-1HAB1.2pm plants turning green was even lower than for hab1-1 ( Fig. 2d,e ). These results indicate that HAB1.1 and HAB1.2 play opposing roles in the regulation of seed germination and post-germination developmental arrest induced by ABA. The HAB1.2 isoform lacks nearly all phosphatase activities To elucidate the regulatory mechanism of HAB1 splicing in response to ABA, we compared the HAB1.1 and HAB1.2 isoforms. A putative nuclear localization signal was detected in the missing 105 amino-acid sequence in the C-terminal portion of HAB1.2 (ref. 29 ; Supplementary Fig. 2a ). Thus, we speculated that the subcellular localization of HAB1.2 maybe altered. First, we tested the subcellular localization of the two isoforms by transiently expressing GFP-HAB1.1 and GFP-HAB1.2 fusion proteins driven by the CaMV 35S promoter in Nicotiana benthamiana leaf cells. As expected, HAB1.1 was localized in both the cytoplasm and nucleus ( Fig. 3a ). To our surprise, HAB1.2 was also localized in both the cytoplasm and nucleus ( Fig. 3a ). Expression of individual HAB1 isoforms was confirmed by immunoblot using anti-green fluorescent protein (GFP) antibody ( Supplementary Fig. 3 ). Cytoplasmic and nucleus localization of HAB1.2 was also validated when it was expressed in hab1-1 plants ( Supplementary Fig. 4 ). These results suggest that HAB1.2 has a similar localization with HAB1.1 in Arabidopsis . 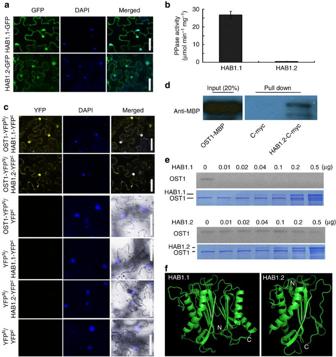Figure 3: The two HAB1 isoforms have different levels of phosphatase activity and different effects on OST1 activity. (a) Subcellular localization analysis of HAB1.1 and HAB1.2 in the transient transformation ofN. benthamianaleaf cells. Scale bar, 20 μm. (b) Comparison of the phosphatase activity of the two HAB1 isoformsin vivo.Recombinant HAB1.1 and HAB1.2 proteins were purified inE. coliand 100 ng proteins were used for the phosphatase activity assay. The s.d. of three experiments is shown using error bars. (c) Interaction between the HAB1 isoforms and OST1 in a BiFC assay. The HAB1.1-YFPCand HAB1.2-YFPCwere co-transformed intoN. benthamianaleaf cells with OST1-YFPN. At 48 h after transformation, the transformed leaves were stained with 4,6-diamidino-2-phenylindole (DAPI) for 15 min and used for the fluorescence observation. (d) Pull-down assay of the HAB1.2 and OST1 interaction. Equal amounts of the purified OST1–MBP fusion protein was added to tubes containing c-Myc-Agarose beads and c-Myc-Agarose beads plus HAB1.2-c-Myc protein, respectively. Anti-MBP antibody was used to detect the HAB1.2–OST1 interaction. (e) Effects of HAB1.1 and HAB1.2 on OST1 phosphorylation activity. OST1 protein was mixed with different concentrations of HAB1 isoforms for 30 min in kinase buffer and the auto-phosphorylation activity of OST1 was detected using phosphorimager. (f) Structures of the HAB1 isoforms predicted by the ESyPred3D software. Figure 3: The two HAB1 isoforms have different levels of phosphatase activity and different effects on OST1 activity. ( a ) Subcellular localization analysis of HAB1.1 and HAB1.2 in the transient transformation of N. benthamiana leaf cells. Scale bar, 20 μm. ( b ) Comparison of the phosphatase activity of the two HAB1 isoforms in vivo. Recombinant HAB1.1 and HAB1.2 proteins were purified in E. coli and 100 ng proteins were used for the phosphatase activity assay. The s.d. of three experiments is shown using error bars. ( c ) Interaction between the HAB1 isoforms and OST1 in a BiFC assay. The HAB1.1-YFP C and HAB1.2-YFP C were co-transformed into N. benthamiana leaf cells with OST1-YFP N . At 48 h after transformation, the transformed leaves were stained with 4,6-diamidino-2-phenylindole (DAPI) for 15 min and used for the fluorescence observation. ( d ) Pull-down assay of the HAB1.2 and OST1 interaction. Equal amounts of the purified OST1–MBP fusion protein was added to tubes containing c-Myc-Agarose beads and c-Myc-Agarose beads plus HAB1.2-c-Myc protein, respectively. Anti-MBP antibody was used to detect the HAB1.2–OST1 interaction. ( e ) Effects of HAB1.1 and HAB1.2 on OST1 phosphorylation activity. OST1 protein was mixed with different concentrations of HAB1 isoforms for 30 min in kinase buffer and the auto-phosphorylation activity of OST1 was detected using phosphorimager. ( f ) Structures of the HAB1 isoforms predicted by the ESyPred3D software. Full size image HAB1 phosphatase activity plays an essential role in inactivating the kinase activity of OST1 (ref. 17 ). HAB1.2, truncated at its C terminus, carries an incomplete PP2ase catalytic domain ( Supplementary Fig. 2a ). This finding led us to question whether the phosphatase activity of HAB1.2 is different from that of HAB1.1. To answer this question, we fused HAB1.1 and HAB1.2 in-frame with maltose-binding protein (MBP) to create HAB1.1-MBP and HAB1.2-MBP fusion proteins, and the phosphatase activity of the two HAB1 isoforms was compared in vitro using the phosphopeptide RRA(pT)VA as a substrate. As shown in Fig. 3b , the PP2ase activity of HAB1.1 was 26.79 μm min −1 mg −1 , compared with only 0.47 μm min −1 mg −1 for HAB1.2. Thus, the overall PP2ase activity of HAB1.2 was reduced by 98.5% ( Fig. 3b ). These results indicate that HAB1 AS regulates the catalytic activity of HAB1. HAB1.2 interacts with OST1 but cannot dephosphorylate OST1 Since HAB1.2 lacks a complete PP2C catalytic domain, we speculated that HAB1.2 may have altered activity towards OST1. To test this, we fused full-length OST1 in-frame to the N terminus of YFP to generate OST1-YFP N , and HAB1.1 or HAB1.2 to the C terminus of YFP to generate HAB1.1-YFP C or HAB1.2-YFP C . These constructs were coexpressed in N. benthamiana leaf cells. As expected, HAB1.1 interacted with OST1 in both the cytoplasm and nucleus ( Fig. 3c ). Surprisingly, HAB1.2 also physically interacted with OST1 ( Fig. 3c ). To confirm the physical interaction between HAB1.2 and OST1, we expressed two fusion proteins, HAB1.2-MBP in E. coli and OST1-Myc using the TNT T7/T3-coupled Wheat germ extract system. Using these fusions, the interaction of HAB1.2 with OST1 was confirmed in an in vitro pull-down assay ( Fig. 3d ). Our results suggest that the missing 105 amino acids at the C terminus of HAB1.2 do not affect its interaction with OST1. Next, we examined whether the HAB1.2 isoform affects OST1 kinase activity. To this end, we performed an in vitro kinase assay to examine the autophosphorylation level of OST1 in the presence of HAB1.1 or HAB1.2. As shown in Fig. 3e , HAB1.1 effectively dephosphorylated OST1; by contrast, HAB1.2 did not affect the phosphorylation of OST1 ( Fig. 3e ), indicating that the 105 amino acids at the C-terminal end of HAB1 are required for the dephosphorylation of OST1. To investigate whether the lack of a C terminus in HAB1 changes the protein’s structure, we obtained three-dimensional (3D) structures for both HAB1.1 and HAB1.2 using the ESyPred3D software [30] . As shown in Fig. 3f , the structure of HAB1.1 was similar to that described in a previous report [10] . Surprisingly, the predicted structure of HAB1.2 was dramatically changed. In particular, two α-helices located at the C terminus of HAB1.1 were predicted to be missing in HAB1.2, and the overall structure of HAB1.2 was more flexible than HAB1.1. Notably, the model suggests that the catalytic cleft of HAB1.1 was missing from the HAB1.2 isoform, and the loop region (the region adjacent to the W385-containing HAB1 PYL-interaction site) of the protein was also affected, indicating that HAB1.2 may be inactive in both steps of OST1 inactivation. On the basis of these data we suggest that the HAB1.2 isoform functions as a dominant-negative regulator of ABA signalling. A mutation in RBM25 alters HAB1 AS and ABA sensitivity RBM proteins are important regulators in pre-mRNA splicing, and many RBM proteins are involved in the regulation of development and stress response [28] . In humans, HsRBM25 is a novel splicing factor that regulates pre-mRNA AS of an apoptotic factor Bcl-x producing the two isoforms, which have opposing roles during apoptosis [31] . We therefore hypothesized that the HsRBM25 homologue in Arabidopsis is involved in HAB1 AS. A blast search using the HsRBM25 cDNA sequence identified the Arabidopsis gene (At1g60200) as the closest homologue ( Supplementary Fig. 2c ). We obtained a T-DNA-tagged mutant (SALK_064472) of the gene and found that a mutation in the gene caused altered HAB1 splicing. A T-DNA insertion in the 3′untranslated repeat of the gene completely disrupted RBM25 expression; therefore, the mutant was named rbm25 ( Fig. 4a,b ). Expression analysis showed that the HAB1.2 / HAB1.1 ratio was greatly altered at the germination stage. The HAB1.2 / HAB1.1 ratio was ∼ 0.17 and 0.49 in the absence and presence of ABA, respectively, in the wild type ( Fig. 1d ), whereas in the rbm25 mutant the HAB1.2 / HAB1.1 ratio was increased dramatically to 1.5 and 2.5 in the absence and presence of ABA, respectively ( Fig. 4c,d ). This result demonstrates that RBM25 may regulate the AS of HAB1 . 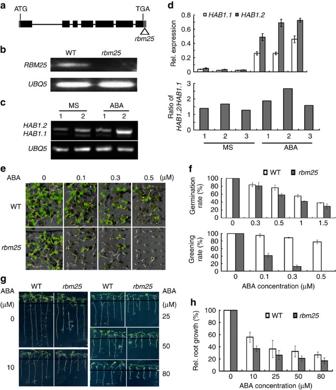Figure 4: A loss of function ofRBM25disturbsHAB1AS and alters ABA sensitivity. (a) Schematic diagram of the T-DNA insertion in therbm25mutant. (b) RT–PCR analysis ofRBM25transcript levels in therbm25mutant. (c) RT–PCR analysis of theHAB1variants inrbm25mutant at 1 and 2 days after germination with or without 100 μM ABA treatment for 3 h.UBQ5was used as a loading control. (d) qRT–PCR analysis of theHAB1variants inrbm25mutant at 1, 2 and 3 days after germination with or without 100 μM ABA treatment for 3 h.GAPDHwas used as an internal control. The values were normalized to that ofGAPDH. The s.d. of three technical replicates is shown using error bars. More than three biological replicates were performed and each gave the similar result. (e) Phenotypic analysis of wild-type (WT) plants and therbm25mutant on MS medium with or without ABA. The pictures were taken 8 days after germination. (f) Comparison of the germination (top) and greening (bottom) rates between WT plants and therbm25mutant. The germination and greening rates were scored 5 and 8 days after germination, respectively. The s.d. of three independent experiments is shown using error bars. (g) Root growth in WT andrbm25plants grown in medium with or without ABA. Five-day-old seedlings from MS medium were transferred to plates with or without ABA and then grown for another 7 days. (h) Quantitative analysis of root growth in WT andrbm25plants. Figure 4: A loss of function of RBM25 disturbs HAB1 AS and alters ABA sensitivity. ( a ) Schematic diagram of the T-DNA insertion in the rbm25 mutant. ( b ) RT–PCR analysis of RBM25 transcript levels in the rbm25 mutant. ( c ) RT–PCR analysis of the HAB1 variants in rbm25 mutant at 1 and 2 days after germination with or without 100 μM ABA treatment for 3 h. UBQ5 was used as a loading control. ( d ) qRT–PCR analysis of the HAB1 variants in rbm25 mutant at 1, 2 and 3 days after germination with or without 100 μM ABA treatment for 3 h. GAPDH was used as an internal control. The values were normalized to that of GAPDH . The s.d. of three technical replicates is shown using error bars. More than three biological replicates were performed and each gave the similar result. ( e ) Phenotypic analysis of wild-type (WT) plants and the rbm25 mutant on MS medium with or without ABA. The pictures were taken 8 days after germination. ( f ) Comparison of the germination (top) and greening (bottom) rates between WT plants and the rbm25 mutant. The germination and greening rates were scored 5 and 8 days after germination, respectively. The s.d. of three independent experiments is shown using error bars. ( g ) Root growth in WT and rbm25 plants grown in medium with or without ABA. Five-day-old seedlings from MS medium were transferred to plates with or without ABA and then grown for another 7 days. ( h ) Quantitative analysis of root growth in WT and rbm25 plants. Full size image We then analysed the response of the rbm25 mutant to ABA. In the absence of ABA, seed germination and cotyledon greening in rbm25 were comparable to that in wild type ( Fig. 4e,f ). However, in the presence of ABA, the rbm25 mutant exhibited substantially increased sensitivity to increasing concentrations of ABA. For example, when germinated on medium supplemented with 0.5 μM ABA, the germination rate of rbm25 was reduced by ∼ 20% at 3 days after stratification ( Fig. 4f ). Notably, rbm25 seedlings were hypersensitive to ABA in cotyledon greening ( Fig. 4f ). With increasing concentrations of ABA, cotyledon greening in rbm25 was severely inhibited and was completely inhibited in the presence of 0.5 μM ABA while the greening rate in wild type was as high as 77.75% ( Fig. 4f ). Root growth in rbm25 seedlings germinated on Murashige and Skoog (MS) medium was also more sensitive to ABA than that in wild type ( Fig. 4g,h ). HAB1.1 overexpression rescues rbm25 ABA hypersensitivity The observation that the HAB1.2 / HAB1.1 ratio in rbm25 was higher than that in wild type led us to question whether the misregulation of HAB1 AS is responsible for the ABA-sensitive phenotype of rbm25 . If this was true, then the overexpression of HAB1.1 may be expected to restore the phenotype of the rbm25 mutant. To answer this question, we expressed the full-length cDNA of HAB1.1 driven by the CaMV 35S promoter in rbm25 mutant plants ( Fig. 5a ) and analysed the HAB1.2 / HAB1.1 ratio and sensitivity of the transgenic lines to ABA during seed germination and post-germination development. As shown in Fig. 5a , HAB1.1 was highly overexpressed in the rbm25 transgenic lines. The HAB1.2/HAB1.1 ratios in the rbm25HAB1.1 lines were substantially reduced compared with that in rbm25 and were even lower than that in wild type ( Fig. 5b ). Importantly, the overexpression of HAB1.1 in rbm25 restored its ABA-sensitive phenotypes, including delayed germination and the post-germinative growth arrest ( Fig. 5c,d ). To avoid unspecific effects due to misexpression of HAB1.1 , we also introduced the HAB1.1 driven by its native promoter into rbm25 mutant and found that the ABA-sensitive phenotype of rbm25 was completely restored ( Supplementary Fig. 5 ). These results suggest that the increased ABA sensitivity of rbm25 was caused by the reduced expression of HAB1.1 and increased HAB1.2 / HAB1.1 ratio. 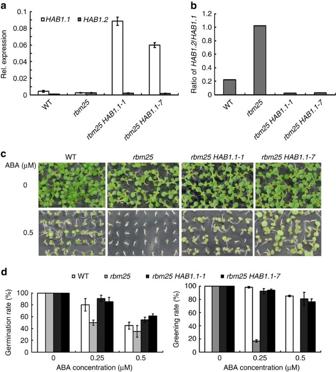Figure 5:HAB1.1overexpression inrbm25rescues the ABA sensitivity ofrbm25. (a) qRT–PCR analysis of theHAB1variants in WT plants,rbm25and two transgenic lines expressing35S::HAB1.1-myc. The s.d. of three technical replicates is shown using error bars. Three biological replicates were performed and each gave the similar result. (b) Quantitative analysis of theHAB1.2/HAB1.1ratio ina. (c) Phenotypic analysis of WT plants, therbm25mutant and two transgenic lines grown on MS medium with or without ABA. The pictures were taken 8 days after germination. (d) Quantitative analysis of the germination and greening rates of WT plants,rbm25and two transgenic lines. The germination and greening rates were scored 5 and 8 days after germination. The s.d. of three independent experiments is shown using error bars. Figure 5: HAB1.1 overexpression in rbm25 rescues the ABA sensitivity of rbm25 . ( a ) qRT–PCR analysis of the HAB1 variants in WT plants, rbm25 and two transgenic lines expressing 35S::HAB1.1-myc . The s.d. of three technical replicates is shown using error bars. Three biological replicates were performed and each gave the similar result. ( b ) Quantitative analysis of the HAB1.2 / HAB1.1 ratio in a . ( c ) Phenotypic analysis of WT plants, the rbm25 mutant and two transgenic lines grown on MS medium with or without ABA. The pictures were taken 8 days after germination. ( d ) Quantitative analysis of the germination and greening rates of WT plants, rbm25 and two transgenic lines. The germination and greening rates were scored 5 and 8 days after germination. The s.d. of three independent experiments is shown using error bars. Full size image Overexpression of RBM25 restores rbm25 phenotypes RBM25 contains seven exons and six introns ( Fig. 4a ), is a single-copy gene and is functionally uncharacterized in Arabidopsis . To assess whether the phenotype of the rbm25 mutant is indeed caused by the loss of function of RBM25 , we transformed rbm25 mutant plants with full-length RBM25 cDNA driven by the CaMV 35S promoter ( Supplementary Fig. 6a ). Six transgenic lines overexpressing RBM25 showed altered ABA sensitivity compared with the rbm25 mutant ( Supplementary Fig. 6b,c ). Two transgenic lines, rbm25RBM25-9 and rbm25RBM25-10 , expressing high levels of RBM25 were analysed further ( Fig. 6a ). First, we examined the effect of RBM25 overexpression on HAB1 AS. qRT–PCR analysis showed that the overexpression of RBM25 greatly reduced the HAB1.2/HAB1.1 ratio ( Fig. 6b ), and, importantly, the HAB1.2/HAB1.1 ratio was completely restored to the wild-type level in the presence of ABA ( Fig. 6b ). Next, we analysed the ABA sensitivity of rbm25RBM25-9 and rbm25RBM25-10 . As shown in Fig. 6c–f , the ABA-sensitive phenotypes of rbm25 during both the germination and post-germination stages were completely restored by the overexpression of RBM25 ( Fig. 6c,d ). Root growth in rbm25RBM25-9 and rbm25RBM25-10 seedlings germinated on the MS medium was also similar to that in wild type in the presence of various concentrations of ABA ( Fig. 6e,f ). On the basis of these results we suggest that RBM25 is responsible for the abnormal AS of HAB1 and increased ABA sensitivity observed in rbm25 . 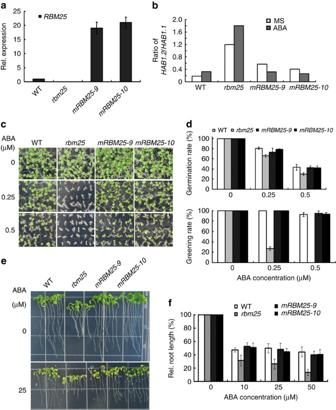Figure 6:RBM25overexpression rescues the ABA sensitivity ofrbm25. (a) qRT–PCR assay ofRBM25expression in WT plants,rbm25and two transgenic lines harbouring35S::RBM25-mycconstruct. RNA was extracted from 7-day-old seedlings germinated on MS medium. The s.d. of three technical replicates is shown using error bars.mRBM25represents the lines overexpressingRBM25in therbm25mutant. (b) Comparison of theHAB1.2/HAB1.1ratio in WT plants,rbm25and two transgenic lines. RNA was extracted from 7-day-old seedlings treated with or without 100 μM ABA for 3 h. (c) Phenotypic analysis of WT andrbm25plants and two transgenic lines grown on MS medium with or without ABA. The pictures were taken 8 days after germination. (d) Comparison of the germination and greening rates among WT plants,rbm25and two transgenic lines. The germination and greening rates were scored 5 and 8 days after germination, respectively. The s.d. of three independent experiments is shown using error bars. (e) Root growth in WT plants,rbm25and two different lines grown in medium with or without ABA. Five-day-old seedlings from MS medium were transferred to plates with or without ABA and grown for another 7 days. (f) Quantitative analysis of root growth in WT plants,rbm25and two transgenic lines in response to ABA. Figure 6: RBM25 overexpression rescues the ABA sensitivity of rbm25 . ( a ) qRT–PCR assay of RBM25 expression in WT plants, rbm25 and two transgenic lines harbouring 35S::RBM25-myc construct. RNA was extracted from 7-day-old seedlings germinated on MS medium. The s.d. of three technical replicates is shown using error bars. mRBM25 represents the lines overexpressing RBM25 in the rbm25 mutant. ( b ) Comparison of the HAB1.2 / HAB1.1 ratio in WT plants, rbm25 and two transgenic lines. RNA was extracted from 7-day-old seedlings treated with or without 100 μM ABA for 3 h. ( c ) Phenotypic analysis of WT and rbm25 plants and two transgenic lines grown on MS medium with or without ABA. The pictures were taken 8 days after germination. ( d ) Comparison of the germination and greening rates among WT plants, rbm25 and two transgenic lines. The germination and greening rates were scored 5 and 8 days after germination, respectively. The s.d. of three independent experiments is shown using error bars. ( e ) Root growth in WT plants, rbm25 and two different lines grown in medium with or without ABA. Five-day-old seedlings from MS medium were transferred to plates with or without ABA and grown for another 7 days. ( f ) Quantitative analysis of root growth in WT plants, rbm25 and two transgenic lines in response to ABA. Full size image RBM25 is ABA-induced and encodes a conserved splicing factor To further understand whether RBM25 is a critical regulator of HAB1 AS in vivo , we first examined the RBM25 expression pattern and features of RBM25. qRT–PCR analysis showed that RBM25 was expressed in various tissues and organs throughout the plant life cycle ( Supplementary Fig. 7a ). Notably, the highest level of expression of RBM25 was detected in seeds, revealing a similar expression pattern to HAB1 ( Fig. 1c ). RBM25 expression was also induced by ABA ( Fig. 7a ); however, the increase in RBM25 expression was much lower than that of HAB1 transcription level under ABA treatment ( Supplementary Fig. 7b ). 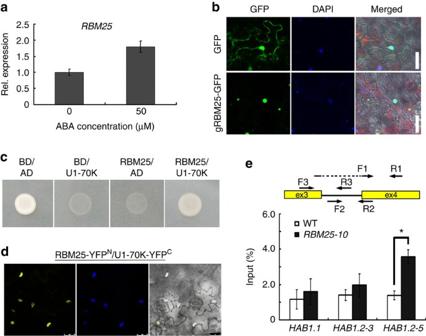Figure 7: RBM25 binding to the last intron ofHAB1. (a)RBM25is induced by ABA slightly. Ten-day-old seedlings germinated on MS medium were treated without or with 100 μM ABA for 3 h, and total RNA was used for qRT–PCR analysis. (b) The construct harbouring gRBM25-GFP was transformed into therbm25plants, and the fluorescence of RBM25-GFP was observed in the leaf cells of 2-week-old seedlings. The nucleus localization of RBM25 was confirmed by DAPI staining. Scale bar, 20 μm. (c,d) Interaction analysis between RBM25 and U1-70K using yeast two-hybrid assay (c) and BiFC analysis (d).(e) RIP assay showing that RBM25 binds to the last intron ofHAB1. Input protein was 10% of total input proteins. The amounts ofHAB1.1, HAB1.2-3andHAB1.2-5fragments were determined by qRT–PCR and normalized to the input.HAB1.1,HAB1.2-3andHAB1.2-5were amplified using the primer pairs of F1/R1, F2 /R2 and F3/ R3, respectively. The s.d. of three biological replicates is shown using error bars (t-test, *P<0.05). Figure 7: RBM25 binding to the last intron of HAB1 . ( a ) RBM25 is induced by ABA slightly. Ten-day-old seedlings germinated on MS medium were treated without or with 100 μM ABA for 3 h, and total RNA was used for qRT–PCR analysis. ( b ) The construct harbouring gRBM25-GFP was transformed into the rbm25 plants, and the fluorescence of RBM25-GFP was observed in the leaf cells of 2-week-old seedlings. The nucleus localization of RBM25 was confirmed by DAPI staining. Scale bar, 20 μm. ( c , d ) Interaction analysis between RBM25 and U1-70K using yeast two-hybrid assay ( c ) and BiFC analysis ( d ). ( e ) RIP assay showing that RBM25 binds to the last intron of HAB1 . Input protein was 10% of total input proteins. The amounts of HAB1.1, HAB1.2-3 and HAB1.2-5 fragments were determined by qRT–PCR and normalized to the input. HAB1.1 , HAB1.2-3 and HAB1.2-5 were amplified using the primer pairs of F1/R1, F2 /R2 and F3/ R3, respectively. The s.d. of three biological replicates is shown using error bars ( t -test, * P <0.05). Full size image Arabidopsis RBM25 encodes an RNA-binding protein that contains an RBM at its N-terminal end and a Pro-Trp-Ile (PWI) motif at its C terminus ( Supplementary Fig. 8a ). The sequence shows strong similarity to HsRBM25 ( Supplementary Fig. 8b,c ), a pre-mRNA splicing factor [31] . There is only a single copy of RBM25 in the Arabidopsis genome, and its homologues are ubiquitously expressed in eukaryotes ( Supplementary Fig. 8d ). Subcellular localization analysis by expressing the genomic RBM25-GFP in Arabidopsis leaf cells showed that RBM25 was exclusively localized in the nucleus ( Fig. 7b ) [32] . The nucleus localization of RBM25 was confirmed by transiently expressing full-length RBM25 cDNA fused in-frame with GFP at the N-terminal end in N. benthamiana ( Supplementary Fig. 9 ). To further examine whether Arabidopsis RBM25 functions as a splicing factor, we assessed the interaction between RBM25 and U1 small nuclear ribonucleoprotein 70 K (U1-70K), which functions in the AS of nuclear pre-mRNAs [33] . Yeast two-hybrid analysis revealed that RBM25 interacted with U1-70K ( Fig. 7c ). We then used the BiFC assay to confirm the interaction between RBM25 and U1-70K in vivo . As shown in Fig. 7d , when RBM25-YFP N and U1-70K-YFP C fusion proteins were transiently coexpressed in N. benthamiana leaf cells, strong YFP fluorescence was observed in the nucleus ( Fig. 7d ), whereas no fluorescence was detected when RBM25-YFP N was coexpressed with empty YFP C ( Supplementary Fig.10 ). These results indicate that RBM25 is a potential splicing factor. RBM25 binding to HAB1 pre-mRNA As RBM25 is a splicing factor and appears to regulate the ratio of HAB1.2/HAB1.1 , we then attempted to examine whether RBM25 binds to HAB1 pre-mRNA directly. To this end, we performed an RNA chromatin immunoprecipitation (RNA-ChIP) assay to test in vivo binding of RBM25 to HAB1 pre-mRNAs using an rbm25 transgenic line expressing RBM25-myc in the presence of ABA. Three pairs of primers spanning the third intron (F1 and R1), the 3′ selection site in the HAB1.2 transcript (F2 and R2) and the 5′ selection site in HAB1.2 (F3 and R3) were used. Anti-myc immunoblot showed that the amount of HAB1.1 and HAB1.2-3′ mRNA fragments immunoprecipitated by RBM25 in the RBM25 - myc transgenic plants was not significantly altered compared with that in the wild-type control ( Fig. 7e ). By contrast, the abundance of HAB1.2-5′ mRNA fragments was twofold higher than that in wild type. On the basis of this result we suggest that RBM25 can bind to the 5′ selection site in the third intron of HAB1 pre-mRNA. To further test for in vitro binding of RBM25 to HAB1 pre-mRNA, we performed electrophoretic mobility shift assays (EMSA) with the RBM25–MBP recombinant protein. Band shifts were clearly detected when the probe of HAB1 pre-mRNA containing the last intron was incubated with the RBM25–MBP protein, and the binding can be inhibited by the competitive probe ( Supplementary Fig. 11a ). By contrast, the binding ability of RBM25 to HAB1 pre-mRNA was greatly reduced when the nucleotides ( Fig. 2a ) at the 5′ splice site in the third intron were mutated (from Gg to At; Supplementary Fig. 11b ). On the basis of these data we suggest that RBM25 can bind HAB1 pre-mRNA at the last intron directly. The central role of group A PP2Cs in ABA signalling was first identified in the early 1990s, and research on the molecular and physiological functions of PP2Cs has accelerated over the past two decades. The last several years have been very fruitful in terms of elucidating the molecular mechanism of PYL-controlled PP2C activity [5] , [11] , [12] , [13] , [14] . However, until now, no study has investigated the mechanisms underlying PP2C activity regulation at the post-transcriptional level. Here we identified the HAB1 splice variant HAB1.2 at both the mRNA and protein levels. We demonstrated that HAB1 AS represents a key mechanism for the regulation of OST1 activity and ABA signalling. Our work also identified an RNA-recognition motif-containing protein, RBM25, as a potential regulator of HAB1 AS and ABA-mediated post-germination growth arrest in Arabidopsis . The full-length transcript HAB1.1 and HAB1.1 isoform have been extensively studied, whereas HAB1.2 mRNA is produced by HAB1 pre-mRNA AS with retention of the last intron and encodes a truncated protein lacking 105 amino acids at the C terminus, resulting in a partial catalytic domain ( Fig. 1b and Supplementary Fig. 2a ). Although the transcript levels of HAB1.1 and HAB1.2 varied greatly among different organs and developmental stages, the HAB1.2/HAB1.1 ratio was relatively stable, including during seed germination and post-germinative growth ( Fig. 1c,d ). Interestingly, the HAB1.2/HAB1.1 ratio was substantially increased when seeds were treated with ABA ( Fig. 1d ). It appears that a high HAB1.2/HAB1.1 ratio is correlated with delayed seed germination and a post-germination developmental arrest; therefore, the HAB1.2 splice variant may facilitate the ABA-induced germination delay and post-germinative growth arrest. Thus, the role of HAB1.2 is clearly opposite to that of HAB1.1 , which positively modulates early development in response to ABA [16] . Our genetic evidence that the overexpression of HAB1.1 and HAB1.2 in hab1-1 reduced or increased ABA sensitivity during seed germination and post-germinative development, respectively ( Fig. 2 ), supports opposing roles for the two splice variants of HAB1 . Further proof for the opposing roles of the two splice variants comes from the observation that the overexpression of HAB1.1 in rbm25 containing high levels of HAB1.2 produced less severe phenotypes than the rbm25 plants ( Fig. 5 ). Therefore, HAB1 AS plays a crucial role in regulating HAB1 expression and its phosphatase activity during seed germination and post-germination development in response to ABA. Despite bioinformatic predictions that among the nine PP2C genes both HAB1 and ABI2 undergo pre-mRNA AS (TAIR), our results show that only HAB1 undergoes AS ( Supplementary Fig. 1 ). Still, we cannot exclude the possibility that AS of the other eight PP2Cs occurs during other developmental stages or in other tissues under conditions of abiotic stress. Further study will be required to elucidate whether AS or other types of post-transcriptional regulation exist to regulate PP2C expression and activity. However, our work provides the first indication of the post-transcriptional regulation of PP2C expression and phosphatase activity in ABA signalling and plant responses to ABA. Previously, it was shown that the nine PP2Cs differ in their subcellular localization [11] , [29] , [34] and interactions with PYLs [5] , [12] , [13] , [29] . Our findings suggest that the regulatory mechanisms of PP2Cs are more complex than previously thought, and the post-transcriptional regulation of PP2C expression adds another layer of complexity to ABA signalling and plant adaptation to stress. Moreover, there are 74 PP2Cs in Arabidopsis that are involved in various cellular processes [35] . To the best of our knowledge, no report has demonstrated the control of PP2C activity by AS. Therefore, our research sheds new light on the regulation of PP2C activity in plants. The splice variant HAB1.2 encodes a truncated protein lacking 105 amino acids at its C terminus, and the HAB1.2 isoform contains an incomplete catalytic domain ( Fig. 1b and Supplementary Fig. 2a ). Since the catalytic domain of HAB1 is essential for the dephosphorylation of SnRK2.6, it is conceivable that HAB1.2 lacks phosphatase activity and fails to dephosphorylate SnRK2.6 ( Fig. 3e ). This result is not surprising because we found that the lack of 105 amino acids at the C terminus of HAB1 causes dramatic changes in the secondary structure of HAB1.2 ( Fig. 3f ). Protein–protein interaction assays revealed that HAB1.2 retains its ability to physically interact with SnRK2.6/OST1 ( Fig. 3c,d ). It is likely that HAB1 interacts with SnRK2.6 at its N terminus because of the relatively stable structure of the N-terminal section of the protein. However, our functional studies clearly demonstrate that the physical binding of HAB1.2 to SnRK2.6 did not block the access of substrates to SnRK2.6 because HAB1.2 overexpression caused ABA-hypersensitive phenotypes ( Fig. 2 ). These results suggest that SnRK2.6 and ABA signalling remained activated and also confirm that HAB1.2 functions as a positive regulator of ABA signalling. Our findings reveal the opposite roles of the HAB1.1 and HAB1.2 isoforms in ABA signalling (that is, as an on/off switch). Thus, the immediate question is how this occurs and what the physiological role in plant adaptation is. It is known that in the absence of ABA, the 1:1 interaction of HAB1 and SnRK2.6 switches ABA signalling off [10] . In contrast, the binding of HAB1 by PYLs at the same ratio and in the presence of ABA turns ABA signalling on [5] , [6] , [7] . However, it has long been noticed that in the presence of ABA, PYL expression is decreased, while HAB1 and SnRK2.6 expression is greatly increased [14] . Taking the ratios of PYLs and HAB1 or HAB1 and SnRK2.6 into account, the decrease in PYLs and increases in HAB1 and SnRK2.6 under prolonged ABA treatment would promote the interaction of HAB1 and SnRK2.6 and rapidly switch ABA signalling off. This may be a good adaptive strategy for plants in response to ABA treatment and water stress because the immediate switching off of ABA signalling would allow plants to avoid overreacting to their environment. However, plants frequently encounter short- or long-term stress instead of instant water stress under natural conditions [36] . Obviously, the immediate attenuation of ABA signalling is not suitable for the adaptation of plants to prolonged stress. The identification of the HAB1.2 isoform may explain how SnRK2.6 can remain active while ABA signalling is kept on. During exposure to prolonged stress and ABA, the level of HAB1.2 , produced through HAB1 AS, was greatly increased compared with that of HAB1.1 ( Fig. 1d ). Thus, in addition to its interaction with HAB1.1, SnRK2.6 can interact with HAB1.2 resulting in the maintenance of SnRK2.6 activity and constant activation of ABA signalling ( Fig. 3c–e ). Thus, it is conceivable that the molecular function of the HAB1.2 isoform is to compete with HAB1.1 for interaction with SnRK2.6, and to maintain the active form of SnRK2.6 to prevent the kinase and ABA signalling from being switched off ( Fig. 8 ). 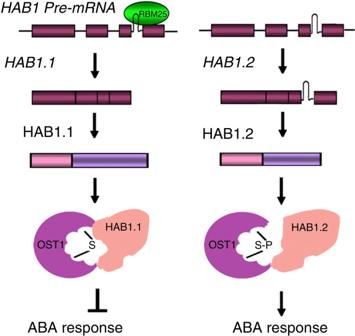Figure 8: A model of RBM25-mediatedHAB1alternative splicing by which HAB1 splice variants control ABA signalling. We suggest that RBM25 can bind to the last intron ofHAB1pre-mRNA and regulate the alternative splicing ofHAB1producing two splice variantsHAB1.1andHAB1.2.HAB1.1contains four exons and encodes a protein, which interacts with the SnRK2.6/OST1 and inhibits its kinase activity switching the ABA signalling off;HAB1.2contains four exons and the last intron and encodes a truncate protein lacking 105 amino acids at the C-terminal end. HAB1.2 still interacts with the SnRK2/OST1 but cannot inhibit its kinase activity, thereby keeping ABA signalling on. Figure 8: A model of RBM25-mediated HAB1 alternative splicing by which HAB1 splice variants control ABA signalling. We suggest that RBM25 can bind to the last intron of HAB1 pre-mRNA and regulate the alternative splicing of HAB1 producing two splice variants HAB1.1 and HAB1.2 . HAB1.1 contains four exons and encodes a protein, which interacts with the SnRK2.6/OST1 and inhibits its kinase activity switching the ABA signalling off; HAB1.2 contains four exons and the last intron and encodes a truncate protein lacking 105 amino acids at the C-terminal end. HAB1.2 still interacts with the SnRK2/OST1 but cannot inhibit its kinase activity, thereby keeping ABA signalling on. Full size image In light of the above results, the regulation of HAB1 AS is of great importance for understanding the regulation of ABA signalling and plant-adaptive responses. RBM25 has been established as a novel splicing factor in humans. HsRBM25 regulates the AS of the apoptosis factor Bcl-x to produce the pro-apoptotic Bcl-xS and anti-apoptotic Bcl-xL isoforms, which have opposite roles in the regulation of apoptosis [31] . On the basis of this work, we suggest that Arabidopsis RBM25 regulates HAB1 AS ( Fig. 7 and Supplementary Fig. 8b,c ). Arabidopsis RBM25 shares high sequence identity to HsRBM25 and possesses all of the features of a splicing factor: it is a nuclear protein ( Fig. 7b and Supplementary Fig. 9 ), can physically interact with the pre-spliceosomal component U1-70K ( Fig. 7c,d ) and appears to be capable of binding to the third intron of the HAB1 pre-mRNA and regulating the AS of HAB1 ( Fig. 7e and Supplementary Fig. 11 ). Therefore, we suggest RBM25 may be a new splicing factor for regulation of HAB1 AS in Arabidopsis . Several lines of evidence support the regulatory role of RBM25 in HAB1 AS. First, RBM25 and HAB1 are coexpressed in multiple tissues and organs, with high levels of expression in mature seeds ( Supplementary Fig. 7a ); both HAB1 and RBM25 genes were induced by ABA ( Fig. 7a and Supplementary Fig. 7b ). The coexpression of RBM25 and HAB1 indicates that they may be functionally related. Second, a loss-of-function mutation in RBM25 resulted in a great increase in the ratio of HAB1.2/HAB1.1 and ABA-hypersensitive phenotypes ( Fig. 4 ). Conversely, the overexpression of RBM25 in the rbm25 mutant background restored HAB1.2/HAB1.1 and plant ABA responses to normal levels ( Fig. 6 ). The fact that the expression of RBM25 was directly correlated to the HAB1.2/HAB1.1 ratio and ABA sensitivity of plants suggests that RBM25 modulates seed germination and post-germinative growth in response to ABA by regulating the AS of HAB1 . Thus, we suggest that RBM25 regulates HAB1 AS, yielding functionally opposing HAB1.2 and HAB1.1 isoforms to control the subsequent switching off and on of the ABA signalling pathway and to mediate adaptive responses ( Fig. 8 ). An immediate question is how the ratio of HAB1.2/HAB1.1 may be controlled through RBM25 in response to ABA. It is known that HAB1 expression is highly induced by ABA [16] . We noticed that the absolute level of HAB1.1 was still much higher than HAB1.2 , although the HAB1.2/HAB1.1 ratio was markedly increased in response to ABA treatment ( Fig. 1 ). We suggest that ABA can promote HAB1 AS by increasing RBM25 expression ( Fig. 7a ). Then, the next key question is how the high HAB1.2/HAB1.1 ratio is achieved? Our results revealed that the extent of the induction of RBM25 gene expression was much lower than that of HAB1 , although both genes are induced by ABA ( Fig. 7a and Supplementary Fig. 7b ). Thus, it is possible that when beyond the capacity of RBM25 in splicing of HAB1 pre-mRNAs (that is, increased transcription level) the rest of HAB1 pre-mRNAs remain unspliced, resulting in relatively increasing levels of HAB1.2 and subsequent higher HAB1.2 / HAB1.1 ratio. Therefore, the levels of ABA and treatment duration may control the levels of HAB1 pre-mRNA, RBM25 expression and the binding activity of RBM25 to HAB1 pre-mRNAs that may fine-tune the HAB1.2/HAB1.1 ratio, ABA signalling and subsequent plant responses. It is well known that the regulation of AS of a given gene is complex. Although RBM25 is responsive to ABA and is capable of binding HAB1 pre-mRNA, it is conceivable that many other proteins are involved in HAB1 AS, such as proteins that may facilitate RBM25 binding to HAB1 pre-mRNA or activate HAB1 pre-mRNA AS. It is also likely that the RBM25-containing splicing complex regulates AS of other genes. Further study of the RBM25-containing splicing complex will decipher the mechanism by which AS of HAB1 and other genes are regulated during development and plant response to abiotic stress. Plant materials and growth conditions A. thaliana ecotype Columbia-0 was used in this study. Seeds were surface-sterilized with 50% bleach, washed three times with sterile water and then grown on MS medium (Sigma-Aldrich, St Louis, MO, USA) containing 2% (w/v) sucrose and 0.3% phytogel (Sigma-Aldrich). The plates were stratified in darkness for 2 days at 4 °C and then transferred to a chamber set at 22 °C under a 16 h of light/8 h of dark photoperiod. After 2 weeks, the seedlings were potted in soil and placed in a growth chamber. Expression assay Seeds germinated on MS in 1, 2 and 3 days were treated with or without 100 μM ABA for 3 h. Total RNA was isolated using Trizol reagent (Life Technologies, Carlsbad, CA, USA) and treated with DNase I (Promega, Madison, WI, USA). qRT–PCR was performed. The relative expression levels of the target genes were calculated by the equation Y =2 C t ( C t is the difference in C t between the target and control products; that is, C t = C tHAB1.1 − C tGAPC ). The primers used for reverse transcription and PCR are listed in Supplementary Table 1 . Germination and root growth assay For phenotypic analysis in the presence of ABA, the MS medium was supplemented with 1% sucrose and different concentrations of ABA. Seeds ( ∼ 80) were surface-sterilized and then plated (three plates per treatment). The plates with seeds were stratified at 4 °C for 2 days and then transferred to a chamber at 22 °C. Seedlings with elongated radicles were counted every 24 days. For the root growth assay, seeds were plated on the MS medium and after 5 days the seedlings were transferred to plates containing different concentrations of ABA [37] . Root growth was then measured after 7 days. Vector construction and plant transformation Binary vectors carrying 35S::6 × myc-AtRBM25 were generated. The full-length 2.7-kb AtRBM25 cDNA fragment was amplified from cDNA and verified by sequencing. The PCR fragment was inserted into the Kpn I– Sac I sites in pCAMBIA1300, in which transgene expression is driven by the CaMV 35S promoter. For the overexpression of HAB1.1, the 1.4-kb length of HAB1.1 was amplified from cDNA and verified by sequencing. The PCR fragment was inserted into the Kpn I– Sac I sites of pCAMBIA1300. For the overexpression of HAB1.2, the 1.6-kb length of HAB1.2 was amplified and cloned into the T-vector. The GG nucleotide acids were mutated to AT using a point mutation kit and then the HAB1.2 fragment containing the two point mutations was inserted into the Kpn I– Sac I sites of pCAMBIA1300. Each construct was transformed into Agrobacterium tumefaciens strain GV3101 and then introduced into rbm25 . T1 plants were selected on MS medium containing hygromycin B. Subcellular localization For transient expression in N. benthamiana leaf cells, 35S::GFP-RBM25, 35S::GFP-HAB1.1 and 35S::GFP-HAB1.2 were constructed using standard molecular biological techniques and Gateway technology (Life Technologies) as described below. To construct 35S::GFP-RBM25, full-length RBM25 was amplified and inserted into the Kpn I– Sac I sites of the binary vector pEZR(K)-LC (ref. 38 ). The open reading frames of HAB1.1 and HAB1.2 were amplified and the fragments were first cloned into pDONR207 and then into pGWB6 (ref. 39 ) to generate 35S::GFP-HAB1.1 and 35S::GFP-HAB1.2, respectively. The primers used for reverse transcription and PCR are listed in Supplementary Table 1 . The constructs were injected into 3- to 4-week-old N. benthamiana plants as described [39] . At 2–4 days after injection, fluorescence was observed with a Zeiss LSM510 confocal microscope (Jena, Germany). BiFC analysis The binary vectors used in this experiment were the reconstructed pEarleyagte201-YN and pEarleygate202-YC vectors described in ref. 40 . RBM25 was cloned into pEarleyagte201-YN to generate AtRBM25-YFP N , while U1-70K was cloned into pEarleygate202-YC to generate U1-70K-YFP C . To test the interaction of OST1 with HAB1.1 and HAB1.2, OST1 was cloned into pEarleygate201-YN to generate OST1-YFP N , while the open reading frame of HAB1.1 or HAB1.2 was cloned into pEarleygate202-YC to generate HAB1.1-YFP C and HAB1.2-YFP C , respectively. The primers used for reverse transcription and PCR are listed in Supplementary Table 1 . Agrobacterium strain GV3101 containing each gene was cultured overnight and the OD600 was adjusted to 0.6–0.8. An equal volume of each culture was mixed together for injection. At 2–4 days after injection, YFP fluorescence was detected with a Zeiss LSM510 confocal microscope. RNA-ChIP assay An RNA-ChIP-IT Kit (53024; Active Motif, Carlsbad, CA, USA) was used in this assay with some modifications. Briefly, 12-day-old seedlings treated with ABA (50 μM) for 3 h were harvested and subjected to 1% (w/v) formaldehyde for crosslinking and then ground to a fine powder. After being suspended in 30 ml of buffer (0.44 M sucrose, 20 mM HEPES-KOH (pH=7.4), 10 mM MgCl 2 , 0.5% Triton X-100, 5 mM dithiothreitol (DTT) and 0.1 mM phenylmethyl sulphonyl fluoride) for 15 min on ice, pellets were obtained by centrifugation. The chromatin-enriched pellets were resuspended in 350 μl of Complete Shearing Buffer AM2 (Active Motif). The chromatin was then sheared with a sonicator (SCIENT2-IID; Xinzhi, China) at 6% power with continuous sonication for 2 s at 9-s intervals for 2 min. The crude nuclear fraction was pelleted by centrifugation at 16,000 g for 5 min at 4 °C and then treated with DNase I to digest contaminating DNA. A 1% aliquot was preserved as an input sample and frozen at −80 °C until the reverse crosslinking step. For immunoprecipitation, 10 μg of chromatin were mixed with 4 μg anti-c-myc antibodies (C3956; Sigma) or rabbit IgG (39357; Active Motif) as a control and pre-washed protein G magnetic beads. The mixtures were incubated on a rotator overnight. After washing the beads four times with Complete RNA-ChIP Wash Buffer (Active Motif), immune complexes were eluted by the addition of 250 μl of Elution Buffer (Active Motif). Following the reversal of crosslinking at 65 °C for 1.5 h, the RNA was purified using Trizol solution and 20 μl of Diethyl pyrocarbonate-treated water were added to elute the immunoprecipitated RNA. DNase I treatment was used to remove any residual DNA within the samples before qRT–PCR. A TransScript Green One-Step qRT–PCR SuperMix Kit (AQ2H; TransGen Biotech Co., Ltd.) was used to analyse the level of enrichment. The HAB-related primers used are described in the Supplemental Materials . For quantitative analysis of RBM25-bound pre-mRNAs, the amount of pre-mRNA in the precipitates was normalized to that 10% input. The percentage of input was calculated as 100 × 2 ( C t of input− C t of IP) × 0.1 (0.1 is the dilution factor; 10% of input was used for quantitative analysis). Kinase assays OST1, HAB1.1 and HAB1.2 were expressed as MBP fusion proteins from the expression vector pMAL-c2x (NEB). The fused protein was purified by the Amylose resin as described by the protocol. Kinase assay was performed according to ref. 17 . Briefly, SnRK2 kinases were pre-incubated with concentrations of HAB1.1 or HAB1.2 in kinase buffer (20 mM Tris, pH 7.8, 20 mM MgCl 2 , 1 mM DTT) for 30 min, and then NaF (10 mM), β-glycerophosphate (25 mM) and 2 μCi ATPγ 32 P (3000 Ci mmol −1 ) were added to a 30-μl final volume and incubated at 25 °C for 60 min. Reactions were terminated by addition of SDS sample buffer and subjected to SDS–PAGE. Gels were subjected to autoradiography using a typhoon Trio instrument (GE Company). PP2C activity assays The PP2C activity was assayed using a serine/threonine phosphatase assay system (Promega) according to the manufacturer’s protocols. MBP (0.1 μM)-fused HAB1.1 and HAB1.2 were reacted with 0.1 mM RRA(pT)VA phosphopeptide substrate in a reaction buffer (50 mM imidazole, pH 7.2, 0.2 mM EGTA, 5 mM MgCl 2 , 0.02% β-mercaptoethanol and 0.1 mg m1 −1 BSA). Electrophoretic mobility shift assays ATPγ 32 P-labelled RNA transcripts for EMSA were transcribed from HAB1 genome DNA with SP6 or T7 polymerase using the MAXIscript Kit (AM1308). EMSA were carried out by using ∼ 0.2 μCi (Perkin-Elmer Corp., NEG507H250UC) of UTP-labelled RNA per reaction. Binding reactions were carried out in binding buffer (10 mM Tris-HCl, pH 7.5, 1.5 mM MgCl 2 , 250 mM KCl, 0.5 mM DTT, 0.5% Triton X-100, Protease inhibitor mix tablet (Complete ULTRA Tablets, Mini, 05892791001, Roche, UK) in a 20-μl total volume, and then incubated at 30 °C for 20 min before loading the samples. Competitor RNA was added at the beginning of the reaction, where indicated. The reactions were resolved on a 5% polyacrylamide gel (Acrylamide:Bis, 40:1) in 1 × Tris-borate-EDTA buffer at 10 V cm −1 . Full scans of the agarose gels and western blots are presented in Supplementary Figs 12–14 . The biological replicates for the experiments are shown in Supplementary Fig. 15 . How to cite this article: Wang, Z. et al. ABA signalling is fine-tuned by antagonistic HAB1 variants. Nat. Commun. 6:8138 doi: 10.1038/ncomms9138 (2015).